Structural and functional features of a collagen-binding matrix protein from the mussel byssus Blue mussels adhere to surfaces by the byssus, a holdfast structure composed of individual threads representing a collagen fibre reinforced composite. Here, we present the crystal structure and function of one of its matrix proteins, the proximal thread matrix protein 1, which is present in the proximal section of the byssus. The structure reveals two von Willebrand factor type A domains linked by a two-β-stranded linker yielding a novel structural arrangement. In vitro , the protein binds heterologous collagens with high affinity and affects collagen assembly, morphology and arrangement of its fibrils. By providing charged surface clusters as well as insufficiently coordinated metal ions, the proximal thread matrix protein 1 might interconnect other byssal proteins and thereby contribute to the integrity of the byssal threads in vivo . Moreover, the protein could be used for adjusting the mechanical properties of collagen materials, a function likely important in the natural byssus. In order to deal with mechanical challenges caused by waves and currents in the intertidal zone, blue mussels ( Mytilus sp.) adhere to various surfaces by the byssus, a unique holdfast structure composed of individual threads attached to a stem. Byssal threads of Mytilus galloprovincialis ( Fig. 1a ) are almost entirely composed of proteins and produced by a specified organ, the mussel foot. Each thread shows three morphologically different parts, a crimped and elastic proximal and a rather smooth and stiff distal section, and an adhesive plaque at the interface to the substratum ( Fig. 1b ). Mechanically, each thread displays gradual properties from proximally elastic to distally stiff [1] , enabling a smooth mechanical transition from soft tissue (the mussel) to hard substrates (for example, rocks) necessary to avoid weak spots upon mechanical loading [2] . Byssus comprises three distinct collagen proteins termed PreCols [3] , surrounded by matrix proteins that differ significantly between the distal and proximal section, and further adhesive and cohesive proteins in the thread cuticle and the adhesive plaque [4] . In the distal section, 96% of the protein content is collagenous with tightly packed and straightly aligned fibrils predominantly made of the collagen PreCol-D [5] , providing stiffness to the thread [6] . In contrast, in the proximal section, the collagens (predominantly PreCol-P [7] ) are more loosely arranged, appearing as spring-like waves [8] ( Fig. 1c ). The overall collagenous content in the proximal section is much lower, with matrix proteins representing 34% of the dry weight [9] ( Fig. 1d ). Some of these matrix proteins have been identified previously, but only assumptions exist concerning their structure and function [9] , [10] , [11] . 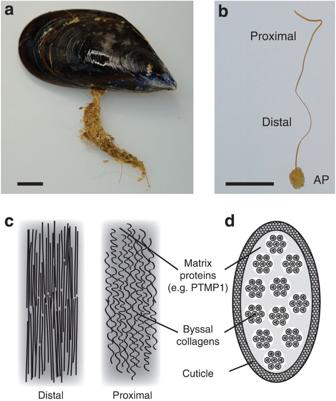Figure 1: The mussel byssus. (a) Blue mussel (M. galloprovincialis) with byssus. Scale bar, 10 mm. (b) Single byssal thread with annotation of the morphologically distinguishable parts, the crimped and elastic proximal and the rather smooth and stiff distal section and the adhesive plaque (AP). Scale bar, 5 mm. (c) Schematic drawing of collagen alignment within individual parts of the thread (longitudinal section). (d) Schematic cross section of a byssal thread showing the distribution of matrix proteins (for example, PTMP1) and collagen fibrils in the core of the proximal thread part. Figure 1: The mussel byssus. ( a ) Blue mussel ( M. galloprovincialis ) with byssus. Scale bar, 10 mm. ( b ) Single byssal thread with annotation of the morphologically distinguishable parts, the crimped and elastic proximal and the rather smooth and stiff distal section and the adhesive plaque (AP). Scale bar, 5 mm. ( c ) Schematic drawing of collagen alignment within individual parts of the thread (longitudinal section). ( d ) Schematic cross section of a byssal thread showing the distribution of matrix proteins (for example, PTMP1) and collagen fibrils in the core of the proximal thread part. Full size image The proximal thread matrix protein 1 (PTMP1) could be localized exclusively in the proximal byssus section and extracted and purified therefrom [11] . The protein appeared to be glycosylated by α- D -manno- or α- d -glucopyranosyl residues. Its protein sequence was determined from the respective cDNA after peptide sequencing and PCR with degenerate primers. It revealed two sequence stretches with homology to the group of von Willebrand factor type A (VWA) domains (Pfam PF00092) with ~25% sequence identity and~50% homology to other members of this group, including the von Willebrand factor A3 domain or the I-domains of integrins. VWA domain containing proteins of the blood plasma or the extracellular matrix are often involved in protein–protein interactions including binding of collagen [12] , [13] , [14] , [15] . In case of the von Willebrand factor, binding to partner proteins like glycoprotein Ib or collagen is dependent on conformational changes upon shear forces [16] , [17] . Many of these VWA domains contain discontiguous and often metal ion coordinating motifs (DXSXS…T…D, with X denoting any amino acid) commonly referred to as metal ion dependent adhesion sites (MIDAS [18] ), and also both VWA domains of PTMP1 (A1 and A2) contain such a MIDAS sequence motif [11] . Here, we present the crystal structure of PTMP1, representing the first molecular structure of a protein from the mussel byssus. The two VWA domains of PTMP1 are interconnected by a rigid two-β-stranded linker yielding a novel structural arrangement. We show that PTMP1 binds collagens with high affinity in vitro , likely involving electrostatic interactions. Thereby, PTMP1 affects assembly, morphology and arrangement of heterologous collagen fibrils, a feature that can be used for distinct applications and likely shapes the mechanical properties of the natural byssus. Crystal structure of PTMP1 To study the structure and function of PTMP1 ( Fig. 2a ), we amplified its DNA sequence from a cDNA library derived from feet of the blue mussel M. galloprovincialis . PTMP1 and several variants thereof were recombinantly produced in Escherichia coli and refolded from inclusion bodies. The full-length protein was crystallized (M.H.S., T.S., C.S. and M.G., manuscript in preparation) resulting in two crystal forms from initial screening and optimization procedures, respectively, which differed in shape and growth rate. Diffraction data sets were obtained from both crystal forms, revealing that the initial crystal belonged to space group C2, and the asymmetric unit contained one PTMP1 molecule ( Supplementary Table 1 ). Surprisingly, crystals from optimization procedures grew faster and appeared to be morphologically different (plate shaped rather than box shaped), they belonged to space group P2 1 , and the asymmetric unit contained two PTMP1 molecules ( Supplementary Table 1 ). Due to the low-sequence identities (~25%) to VWA proteins with known structures, initial phasing attempts by automated molecular replacement failed, but extensive manual searches with various search model combinations finally yielded separate solutions for PTMP1 domains A1 (search model PDB-ID 1AOX [19] ) and A2 (search model PDB-ID 1QC5 (ref. 20) [20] ) in space group C2 (crystal form 1), which were then used for solving the structure of the protein in space group P2 1 (crystal form 2). 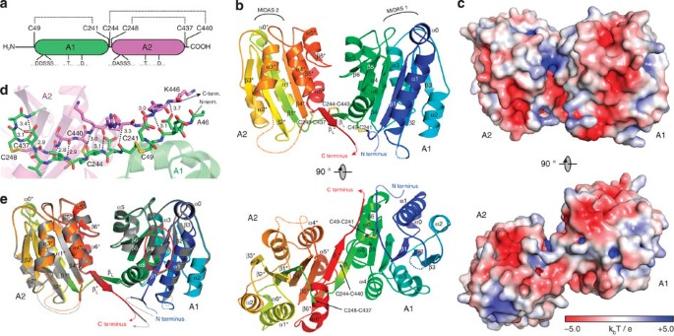Figure 2: Crystal structure of PTMP1. (a) Scheme of the PTMP1 primary structure showing the two VWA domains (A1 and A2), flanked by six cysteines forming three disulphide bonds. The conserved MIDAS motifs are indicated. (b) Crystal structure of PTMP1 in front and bottom view with annotation of the secondary structure elements according to published homologues. Asterisk indicate the respective elements of the A2 domain. The protein is coloured from blue (N terminus) to red (C terminus). Missing residues are indicated by dashed lines. (c) Surface potential of the PTMP1 molecule in front and bottom view coloured from red to blue with a scale of±5kbT e−1. (d) Structural details of the inter-domain linker forming a two-stranded anti-parallel β-sheet. Domain A1 is shown in green, A2 in purple. The disulphide bonds are shown in yellow and positions and lengths (in Å) of the respective H-bonds are indicated. (e) Overlay (RMSD=0.5 Å) of PTMP1 structures solved from diffraction data of crystals with different space groups. The structure from a crystal with space group P21is coloured from blue to red, the structure derived from a crystal with space group C2 is shown in grey. The major difference between the structures in the α6-helix is marked by a red circle. Figure 2: Crystal structure of PTMP1. ( a ) Scheme of the PTMP1 primary structure showing the two VWA domains (A1 and A2), flanked by six cysteines forming three disulphide bonds. The conserved MIDAS motifs are indicated. ( b ) Crystal structure of PTMP1 in front and bottom view with annotation of the secondary structure elements according to published homologues. Asterisk indicate the respective elements of the A2 domain. The protein is coloured from blue (N terminus) to red (C terminus). Missing residues are indicated by dashed lines. ( c ) Surface potential of the PTMP1 molecule in front and bottom view coloured from red to blue with a scale of±5 k b T e −1 . ( d ) Structural details of the inter-domain linker forming a two-stranded anti-parallel β-sheet. Domain A1 is shown in green, A2 in purple. The disulphide bonds are shown in yellow and positions and lengths (in Å) of the respective H-bonds are indicated. ( e ) Overlay (RMSD=0.5 Å) of PTMP1 structures solved from diffraction data of crystals with different space groups. The structure from a crystal with space group P2 1 is coloured from blue to red, the structure derived from a crystal with space group C2 is shown in grey. The major difference between the structures in the α6-helix is marked by a red circle. Full size image The refined structure of PTMP1 in space group P2 1 , solved at a resolution of 1.9 Å ( Supplementary Table 1 ), reveals a monomer with two compactly folded domains ( Fig. 2b ; Supplementary Fig. 1 ). Surface potential calculations by the Adaptive Poisson-Boltzmann Solver (APBS) [21] revealed charge clustering on each domain ( Fig. 2c ), with predominating negative clusters, corresponding to the theoretical isoelectric point of PTMP1 (pI=5.9). The edges of each domain are interconnected by a disulphide bond, which is often observed in VWA domains [22] , [23] , [24] . The two PTMP1 domains are arranged ‘back-to-back’ with a small contact area involving only five potential hydrogen bonds (Q212-E413; K217-S411; K217-I407/N408/A410; H187-E414; T215-S412/Y415). Interestingly, the two PTMP1 domains are nevertheless held in a stable domain arrangement through an extended linker, consisting of the inter-domain region and a C-terminal stretch in anti-parallel orientation. This linker is rigidified by a β-sheet hydrogen pattern and an additional central disulphide bond ( Fig. 2d ). This domain arrangement was observed nearly identically in crystal form 1 (space group C2), despite different crystal contacts ( Fig. 2e ; Supplementary Table 1 ), demonstrating the stability of the relative domain arrangement. The two structures only differ in the length of a single α-helix (α6, numbering of the secondary structure elements according to published VWA domain structures [19] , [20] , [23] , see also Supplementary Fig. 2 ), which is three amino acids longer in crystal form 1 (residues 226–241) than in crystal form 2 (residues 229–241). The two PTMP1 domains A1 and A2 comprise 46% identical and 60% similar residues ( Fig. 3a ), and both domains adopt very similar folds as shown by an overlay of their structures ( Fig. 3b,c ). Furthermore, in contrast to their unique tandem arrangement, the individual domains show a high structural homology to other VWA domains, like the A3 domain of human von Willebrand factor [23] or the I-domains of Integrin α1 and α2 [19] , [20] ( Fig. 3d–f ), despite an only moderate sequence identity ( Supplementary Fig. 2 ). The main differences are an added, small helix α0 in PTMP1 and a shorter α5 compared with integrins. Differences between the two domains within PTMP1 are an extension of the α1–β2 loop by three amino acids (G94-N96), the flexible α3–β4 loop, which could not be fully resolved for A2 (N351–E358 are missing) and the length of helix α6. In addition, the proline-rich amino-terminal expansion of PTMP1 (amino acids 1–45, Fig. 3a ) and the seven carboxy-terminal amino acids (447–453) could not be resolved in the structure, probably indicating high flexibility. 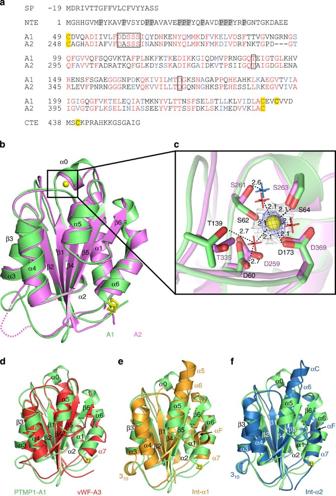Figure 3: Analysis of the PTMP1 VWA domains. (a) Sequence of PTMP1 with annotations of the signal peptide (SP), the terminal expansions (NTE, CTE) and the two VWA domains (A1, A2). The alignment of the domains is shown, with identical and similar amino-acid positions in red and blue, respectively. The amino acids of the putative MIDAS motif are boxed, and the cysteines are highlighted in yellow. Proline residues in the N-terminal expansion are shaded in grey. (b) Overlay (RMSD=0.7 Å) of the two VWA domains of PTMP1 from a Zn-soaked crystal with an indication of the secondary structure elements, the disulphide bonds (yellow sticks) and the Zn2+ion complexed by A1 (yellow sphere). (c) Closeup of (b) displaying structural details of the MIDAS region of A1 and A2 shown as overlay. A1 complexes a Zn2+ion (yellow sphere), indicated by the respective densities (2Fo–Fcmap (contour level 2.0) is shown in grey, anomalous map (contour level 2.5) in blue) and three water molecules (red) complete the zinc-binding site. A2 does not complex a metal ion and features only one water molecule (blue). The respective amino-acid residues and distances (in Å) are indicated. (d) Overlay (RMSD=1.4 Å) of PTMP1 A1 domain (green) and the vWFA3 domain (PDB-ID 1ATZ, red). (e) Overlay (RMSD=0.8 Å) of PTMP1 A1 domain (green) and the I-domain of integrin (Int) α1 (PDB-ID 1QC5, orange). (f) Overlay (RMSD=0.9 Å) of PTMP1 A1 domain (green) and the I-domain of integrin α2 (PDB-ID 1AOX, blue). Figure 3: Analysis of the PTMP1 VWA domains. ( a ) Sequence of PTMP1 with annotations of the signal peptide (SP), the terminal expansions (NTE, CTE) and the two VWA domains (A1, A2). The alignment of the domains is shown, with identical and similar amino-acid positions in red and blue, respectively. The amino acids of the putative MIDAS motif are boxed, and the cysteines are highlighted in yellow. Proline residues in the N-terminal expansion are shaded in grey. ( b ) Overlay (RMSD=0.7 Å) of the two VWA domains of PTMP1 from a Zn-soaked crystal with an indication of the secondary structure elements, the disulphide bonds (yellow sticks) and the Zn 2+ ion complexed by A1 (yellow sphere). ( c ) Closeup of ( b ) displaying structural details of the MIDAS region of A1 and A2 shown as overlay. A1 complexes a Zn 2+ ion (yellow sphere), indicated by the respective densities (2 F o – F c map (contour level 2.0) is shown in grey, anomalous map (contour level 2.5) in blue) and three water molecules (red) complete the zinc-binding site. A2 does not complex a metal ion and features only one water molecule (blue). The respective amino-acid residues and distances (in Å) are indicated. ( d ) Overlay (RMSD=1.4 Å) of PTMP1 A1 domain (green) and the vWFA3 domain (PDB-ID 1ATZ, red). ( e ) Overlay (RMSD=0.8 Å) of PTMP1 A1 domain (green) and the I-domain of integrin (Int) α1 (PDB-ID 1QC5, orange). ( f ) Overlay (RMSD=0.9 Å) of PTMP1 A1 domain (green) and the I-domain of integrin α2 (PDB-ID 1AOX, blue). Full size image To analyse the metal ion binding capacity of the putative MIDAS motifs of PTMP1, crystals were soaked with ZnCl 2 ( Supplementary Table 1 ). Indeed, a Zn 2+ ion was bound to the A1 MIDAS motif (occupancy ~70%), but, surprisingly, not to the A2 motif, which is located on the same side of the PTMP1 molecule ( Fig. 3c ; Supplementary Fig. 3 ). The A2 MIDAS motif is fully conserved and differs from the A1 motif only by an alanine substitution at a non-conserved position not involved in ion binding (DASSS in A2 instead of DDSSS in A1). In the A2 motif, two critical residues (S261 and T335, the latter coordinating a water molecule required for Zn 2+ binding) are slightly turned away from the positions required for metal coordination. There are no obvious restrictions preventing their proper adjustment, though, and this motif thus appears generally capable of ion binding under appropriate conditions. It is tempting to speculate that such conditions could be created through the presence of interacting partner proteins. In the A1 MIDAS motif, the sixfold coordination geometry is consistent with coordinated zinc ions in other proteins [25] . It involves three hydroxyl groups from S62, S64 and D173, respectively, and three water molecules, creating a solvent-exposed metal binding site possibly providing binding possibilities for residues from interacting proteins (see below). The fact that only half of the interaction partners are provided by protein side chains explains the low zinc affinity and occupancy. Furthermore, an additional zinc ion was bound to D50 and H445 (occupancy ~50%) from the central (β L ) and C-terminal β-strand (β L *), respectively, additionally stabilizing the inter-domain linker. Soaking experiments were also performed with MgCl 2 , but binding of magnesium ions to the MIDAS motifs or elsewhere in the PTMP1 molecule could not be observed. Structural stability of PTMP1 To analyse the structural stability of PTMP1, we created deletion variants ΔNΔC (removal of the unstructured N and C termini), A1 and A2 (the isolated PTMP1 VWA domains, Fig. 4a ) that were recombinantly produced and refolded. As predicted from the topology, the structure of two domain constructs is thermally highly stable, as shown by circular dichroism (CD) spectroscopy ( Fig. 4b ). Furthermore, PTMP1 remains monomeric even upon incubation for several hours at 95 °C. The N- and C-terminal expansions of PTMP1 did not exert a significant influence on the structural stability, as shown by spectra and thermal transition curves of the ΔNΔC variant. Strikingly, the isolated PTMP1 domains A1 and A2 showed irreversible aggregation upon heating ( Fig. 4c ). The latter finding further supports the hypothesis of structural stabilization through the linked domains. Chemical unfolding of PTMP1 using guanidine hydrochloride revealed a three-state transition with one apparent intermediate ( Fig. 4d ), and a conformational stability comparable with other proteins with VWA domains [26] . The isolated single VWA domains exhibited an overall lower structural stability against chemical denaturation than the full-length protein. Again, the observed tandem domain arrangement in PTMP1 is a prerequisite for a high stability. 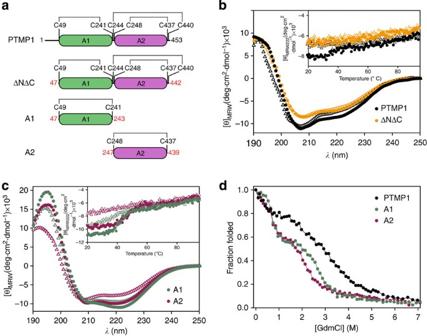Figure 4: Structural stability of PTMP1. (a) Schematic view of PTMP1, the PTMP1 deletion mutant ΔNΔC (PTMP1 amino acids 47–442) and the isolated VWA domains (A1: amino acids 47–243; A2: amino acids 247–439). Mutations of the wild-type protein sequence are highlighted in red. (b) Far ultraviolet CD spectra of PTMP1 (black) and the PTMP1 deletion mutant ΔNΔC (orange) before (circles) and after (triangles) heating. Inset: Thermal transitions of PTMP1 (black) and ΔNΔC (orange) measured by changes of the CD signal at 222 nm. Circles: Heating from 20 to 95 °C; triangles: cooling from 95 to 20 °C. (c) Far ultraviolet CD spectra of PTMP1 and the isolated von VWA domains A1 (green) and A2 (purple) before (circles) and after (triangles) heating. Inset: Thermal transitions of A1 (green) and A2 (purple) measured by changes of the CD signal at 222 nm. Circles: Heating from 20 to 95 °C; triangles: cooling from 95 to 20 °C. (d) Denaturation of PTMP1 (black), A1 (green) and A2 (purple) in the presence of guanidine hydrochloride (GdmCl). All proteins exhibit three-state unfolding with a native state from 0 to ~0.5 M GdmCl, an unfolding intermediate at ~1–2 M GdmCl and an unfolded state above 3 M GdmCl for the isolated domains and above ~5 M for full-length PTMP1. Figure 4: Structural stability of PTMP1. ( a ) Schematic view of PTMP1, the PTMP1 deletion mutant ΔNΔC (PTMP1 amino acids 47–442) and the isolated VWA domains (A1: amino acids 47–243; A2: amino acids 247–439). Mutations of the wild-type protein sequence are highlighted in red. ( b ) Far ultraviolet CD spectra of PTMP1 (black) and the PTMP1 deletion mutant ΔNΔC (orange) before (circles) and after (triangles) heating. Inset: Thermal transitions of PTMP1 (black) and ΔNΔC (orange) measured by changes of the CD signal at 222 nm. Circles: Heating from 20 to 95 °C; triangles: cooling from 95 to 20 °C. ( c ) Far ultraviolet CD spectra of PTMP1 and the isolated von VWA domains A1 (green) and A2 (purple) before (circles) and after (triangles) heating. Inset: Thermal transitions of A1 (green) and A2 (purple) measured by changes of the CD signal at 222 nm. Circles: Heating from 20 to 95 °C; triangles: cooling from 95 to 20 °C. ( d ) Denaturation of PTMP1 (black), A1 (green) and A2 (purple) in the presence of guanidine hydrochloride (GdmCl). All proteins exhibit three-state unfolding with a native state from 0 to ~0.5 M GdmCl, an unfolding intermediate at ~1–2 M GdmCl and an unfolded state above 3 M GdmCl for the isolated domains and above ~5 M for full-length PTMP1. Full size image Collagen-binding properties of PTMP1 It has previously been hypothesized that PTMP1, like other VWA domain containing proteins, binds with and interconnects byssal collagens [9] , [11] . Due to the lack of available PreCol proteins, we analysed binding of heterologous collagens to PTMP1 and its isolated VWA domains using surface plasmon resonance spectroscopy (SPR) [13] , [27] , [28] , since all fibrous collagens show similar structural features. PTMP1 bound immobilized collagen type I with apparent high affinity in the sub-micromolar range as shown by the difference-sensorgram of the collagen-coated versus the reference cell ( Fig. 5a ). Kinetic parameters could be obtained from fits with the 1:1 Langmuir-binding model as described previously for the A3 domain of the human von Willebrand factor [27] . The chosen binding model could be used to fit the data with χ [2] values of generally below 0.5, despite a more probable multivalent-binding scenario. Binding appeared to be mainly dependent on electrostatic interactions since it was inhibited by increasing salt concentrations. As a control, we tested collagen binding to bovine serum albumin (BSA) which equals PTMP1 in monomer size and surface charge. In contrast to PTMP1, BSA bound only weakly to the immobilized collagen, and binding was abolished at higher salt concentrations. Interestingly, the isolated A1 and A2 domains did not significantly bind to a collagen-coated surface ( Fig. 5b ). While, the ΔNΔC deletion mutant exhibited a high-binding capacity, mixing the two isolated domains (which exactly represents the ΔNΔC mutant except of the covalent connection) did not restore high-affinity binding, indicating a strict dependence of collagen binding on the linker-mediated domain arrangement. In addition, the unstructured N- and C-terminal residues might have a regulatory role in collagen binding, since their deletion (ΔNΔC mutant) significantly increased the binding affinity for collagens in SPR analysis. 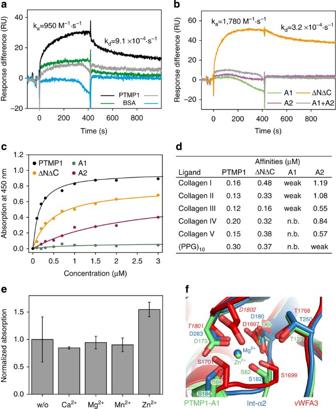Figure 5: Collagen-binding properties of PTMP1. (a) Binding of PTMP1 to immobilized collagen I analysed by SPR spectroscopy (the signal difference between the measurement and reference cell without collagen is shown). As a control, BSA which equals PTMP1 in monomer size and surface charge did not specifically bind collagens. Binding was analysed in the presence of 50 (PTMP1 black, BSA green) and 100 mM sodium chloride (PTMP1 grey, BSA blue). (b) SPR analysis of binding of ΔNΔC (orange), the isolated VWA domains A1 (green), A2 (purple) and a 1:1 mixture thereof (grey) to collagen I. (c) Binding of PTMP1 (black), ΔNΔC (orange) and the isolated VWA domains A1 (green) and A2 (purple) to collagen I analysed by an ELISA-like assay. (d) Apparent affinities (dissociation constants in μM) of PTMP1, ΔNΔC and the isolated domains towards different collagens and the collagen-analog PPG10as determined by ELISA-like experiments (‘weak’ reveals a signal increase with increasing analyte concentration, but the signals do not allow curve fitting; ‘n.b.’, no binding). (e) ELISA-like analysis of PTMP1 (0.1 μM) binding to collagen in the presence of divalent metal ions (mean of three experiments, corrected for background signal±s.d.). (f) Detailed view of the MIDAS regions in the PTMP1 A1 domain (green), the I-domain of integrin α2 (PDB-ID 1AOX) (blue) and the vWFA3 domain (PDB-ID 1ATZ) (red) shown as overlay. PTMP1 A1 coordinates a Zn2+and the Integrin-α2 I-domain a Mg2+ion. The two residues of vWFA3 differing from the regular motif are depicted in italics. Figure 5: Collagen-binding properties of PTMP1. ( a ) Binding of PTMP1 to immobilized collagen I analysed by SPR spectroscopy (the signal difference between the measurement and reference cell without collagen is shown). As a control, BSA which equals PTMP1 in monomer size and surface charge did not specifically bind collagens. Binding was analysed in the presence of 50 (PTMP1 black, BSA green) and 100 mM sodium chloride (PTMP1 grey, BSA blue). ( b ) SPR analysis of binding of ΔNΔC (orange), the isolated VWA domains A1 (green), A2 (purple) and a 1:1 mixture thereof (grey) to collagen I. ( c ) Binding of PTMP1 (black), ΔNΔC (orange) and the isolated VWA domains A1 (green) and A2 (purple) to collagen I analysed by an ELISA-like assay. ( d ) Apparent affinities (dissociation constants in μM) of PTMP1, ΔNΔC and the isolated domains towards different collagens and the collagen-analog PPG 10 as determined by ELISA-like experiments (‘weak’ reveals a signal increase with increasing analyte concentration, but the signals do not allow curve fitting; ‘n.b.’, no binding). ( e ) ELISA-like analysis of PTMP1 (0.1 μM) binding to collagen in the presence of divalent metal ions (mean of three experiments, corrected for background signal±s.d.). ( f ) Detailed view of the MIDAS regions in the PTMP1 A1 domain (green), the I-domain of integrin α2 (PDB-ID 1AOX) (blue) and the vWFA3 domain (PDB-ID 1ATZ) (red) shown as overlay. PTMP1 A1 coordinates a Zn 2+ and the Integrin-α2 I-domain a Mg 2+ ion. The two residues of vWFA3 differing from the regular motif are depicted in italics. Full size image In static ELISA-like assays [28] , PTMP1 bound to a broad range of immobilized soluble heterologous collagens (type I, II, III, IV, V), as well as the collagen-resembling triple-helical peptide (PPG) 10 , with affinities in the sub-micromolar range ( Fig. 5c,d ), as calculated from curve fits according to a one-site binding model. Besides soluble collagen, PTMP1 also bound pre-fibrillized collagens [29] , which has also been shown for the human von Willebrand factor [28] . The isolated A1 and A2 domains both bound collagens in this test, but with much lower affinities than the wild-type protein or the ΔNΔC mutant, which, in contrast to the SPR results, exhibited lower-binding affinity than the full-length protein in this assay. To analyse a putative dependence of collagen-binding on metal ions that are important in case of integrins [14] or matrilins [13] but not in case of the von Willebrand factor [30] , the influence of Ca 2+ , Mg 2+ , Mn 2+ or Zn 2+ was tested. The selective binding of Zn 2+ to the A1 MIDAS motif indicates a contribution to collagen binding. Consistently, collagen binding of PTMP1 was slightly enhanced only in the presence of Zn 2+ , whereas the other metal ions did not exert any apparent influence ( Fig. 5e ). A structural overlay of the collagen-binding MIDAS of integrin α2 (ref. 19) [19] and the respective motif of the human von Willebrand factor A3 domain [23] , which is incapable of binding metal ions, with the A1 domain of PTMP1 reveals that PTMP1 is structurally more related to the integrins than to vWFA3 ( Fig. 5f ), since A1 lacks an aspartate residue present in the MIDAS motif of vWFA3 that is thought to inhibit metal binding [23] . The A2 MIDAS motif, in contrast, did not bind any metal ions tested despite a perfectly conserved MIDAS sequence, and it appears to harbour subtle structural differences to the A1 MIDAS motif (see Fig. 3c ). Strikingly, the A2 domain, like the full-length protein, shows a higher affinity towards collagen in the presence of Zn 2+ , whereas the A1 domain did not show such a Zn 2+ effect (data not shown), in contrast to our previous metal binding results. Since the A2 MIDAS motif provides a binding pocket that should, in principle, allow ion binding, we speculate that collagen can act as a partner protein that completes the ion site, which would explain how the presence of collagen and metal ions influence the binding of each other. In summary, collagen binding of PTMP1 is influenced, but not strictly dependent on the binding of zinc ions. Influence of PTMP1 on collagen assembly and arrangement Since PTMP1 exhibited strong binding to heterologous collagens, we further analysed its potential influence on structure and assembly thereof. Interestingly, the stability of collagen triple helices was not significantly altered in the presence of PTMP1, as shown by thermal unfolding assays employing CD spectroscopy ( Fig. 6a ). Consistently, the secondary structure composition of PTMP1 and collagen type I did not change upon mixing, as indicated by their far ultraviolet CD spectra ( Fig. 6b ). However, PTMP1 interfered with collagen arrangement, as observed by atomic force microscopy (AFM). In the presence of PTMP1, the previously detected alignment of soluble collagens as well as preformed collagen fibrils on mica [31] is significantly impaired ( Fig. 6c ), probably due to electrostatic interactions between PTMP1, collagen and the mica surface. Additionally, the morphology of fibrils reconstituted from soluble collagens in the presence of PTMP1 revealed significant differences to that of collagen fibrils assembled in the absence of PTMP1 as shown by AFM and transmission electron microscopy (TEM) ( Fig. 6d ). Typically, collagen fibrils exhibited a regular and ordered alignment, while the assemblies were thin and more irregular in presence of PTMP1. 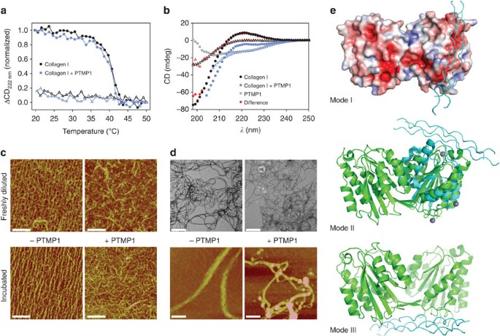Figure 6: Influence of PTMP1 on collagen structure and assembly. (a) Thermal unfolding analysis of collagen I in the absence (black) and presence (blue) of PTMP1 (circles: heating from 20 to 50 °C; triangles: cooling from 50 to 20 °C). The lines are displayed as a guide to the eye. (b) Far ultraviolet CD spectra of collagen I (black), PTMP1 (grey), a 1:1 mixture thereof (blue) and the difference spectra (red) between the respective PTMP1/collagen I mixtures and the PTMP1 spectrum before (circles) and after (triangles) heating. (c) AFM of freshly diluted collagen (upper panels) and collagen fibrils (lower panels) in the absence and presence of PTMP1 as indicated. Scale bars, 0.5 μm. (d) TEM(upper panels) and AFM (lower panels) of fibrils assembled from soluble collagen I in the absence and presence of PTMP1 (as indicated) in solution at pH 8 overnight. Scale bars, TEM: 1 μm; Scale bars, AFM: 0.2 μm. (e) Modelled complexes between PTMP1 and collagen. Mode I: Manual docking of collagen (cyan) on the negatively charged stretch (red) in PTMP1 A1. Mode II: Overlay of PTMP1 (light green) with an integrin I–collagen complex (cyan), showing the binding mode involving the MIDAS metal binding site. Mode III: PTMP1–collagen complex representative for 9 of the 10 top complex predictions obtained with ClusPro52. Figure 6: Influence of PTMP1 on collagen structure and assembly. ( a ) Thermal unfolding analysis of collagen I in the absence (black) and presence (blue) of PTMP1 (circles: heating from 20 to 50 °C; triangles: cooling from 50 to 20 °C). The lines are displayed as a guide to the eye. ( b ) Far ultraviolet CD spectra of collagen I (black), PTMP1 (grey), a 1:1 mixture thereof (blue) and the difference spectra (red) between the respective PTMP1/collagen I mixtures and the PTMP1 spectrum before (circles) and after (triangles) heating. ( c ) AFM of freshly diluted collagen (upper panels) and collagen fibrils (lower panels) in the absence and presence of PTMP1 as indicated. Scale bars, 0.5 μm. ( d ) TEM(upper panels) and AFM (lower panels) of fibrils assembled from soluble collagen I in the absence and presence of PTMP1 (as indicated) in solution at pH 8 overnight. Scale bars, TEM: 1 μm; Scale bars, AFM: 0.2 μm. ( e ) Modelled complexes between PTMP1 and collagen. Mode I: Manual docking of collagen (cyan) on the negatively charged stretch (red) in PTMP1 A1. Mode II: Overlay of PTMP1 (light green) with an integrin I–collagen complex (cyan), showing the binding mode involving the MIDAS metal binding site. Mode III: PTMP1–collagen complex representative for 9 of the 10 top complex predictions obtained with ClusPro [52] . Full size image The crystal structure of recombinant PTMP1 revealed two VWA-like domains interconnected by a highly rigidified linker. Although there are examples of proteins with repeated VWA domains, as for example in collagen VI, cochlin or vitrin [32] , this structural arrangement with a rigid β-sheet-linker is novel. The fact that PTMP1 exhibits only minor inter-domain contacts besides this linker underlines its importance on the stability of this domain arrangement, observed in two different crystal forms of the protein. In addition, both individual domains are structurally less stable than the connected ones. A functional role of the linker as a molecular ligament or even hinge is plausible, since binding of collagen is highly dependent on the presence of the linker and the topology of the two VWA domains, with the individual domains showing only little collagen-binding affinity. PTMP1 binds to different heterologous collagens with high affinities and a dependency of the binding strength on the ionic strength of the environment, and it is thus likely that binding is dominantly mediated by electrostatic interactions. Since PTMP1 exhibits a theoretical isoelectric point of 5.9, electrostatic interactions are likely with basic collagens or, more precisely, with collagen triple-helical regions at pH 7-8. Consistently, the PTMP1 surface potential reveals acidic patches which could be involved in collagen binding. In a first binding mode, collagen positioned along these stripes of negative charges would bind only one VWA domain, from top to bottom ( Fig. 6e , Mode I). Interestingly, the stripe in A1 includes the MIDAS region, and Zn 2+ binding there would generate a positive spot in a negatively charged environment that could act as a specificity marker in this interaction. The collagen-binding mode seen in an integrin I–collagen complex also includes the MIDAS motif, with a Glu from the collagen completing the Zn 2+ coordination [14] . Overlaying PTMP1 with this complex indicates that a similar binding mode is possible. However, collagen is slightly shifted into space provided by the shorter α5 of PTMP1 to avoid clashes with PTMP1 α0 which does not exist in integrin ( Fig. 6e , Mode II). This shift results in a slight tilt of the collagen directing it towards the A2 domain, likely explaining the stronger collagen binding of full-length PTMP1 over the single A1 domain. Due to the repetitive structure of collagens, Zn 2+ could act as anchor in both binding modes for a stick-and-slip interaction observed for other VWA domains. Such interactions would crosslink byssus collagens but allow force-dependent adjustments of the crosslink. Another binding mode predicted by automated docking of the proteins involves the inter-domain linker and possibly the Zn 2+ site in the PTMP1 linker ( Fig. 6e , Mode III). For identifying the correct interaction surface, PTMP1 mutagenesis experiments might not be suitable since many residues are contributing to binding. Although co-crystallization attempts so far failed, this technique, if successful, will allow identifying the interacting residues. Since PTMP1 is also capable of binding triple-helical structures without pronounced electrostatic interactions, like the collagen-resembling triple-helical peptide (PPG) 10 , and the isolated VWA domains bound collagen with much less affinity than when combined, the collagen-binding mode of PTMP1 differs from that of integrins. In addition, the binding differs to that of von Willebrand factor since PTMP1 lacks nearly all of the critical interacting residues of the vWFA3 domain [12] . In the von Willebrand factor and other VWA domain proteins, C-terminal helix and linker act as a switch region between an open and a closed state with low and high affinity for metal and ligand [33] . Interestingly, the C termini of A1 and A2 are coupled in PTMP1, suggesting that a mechanism regulating their ligand affinity could affect both domains concomitantly. However, in light of lack of shear dependent collagen binding in our SPR experiments (data not shown), it remains enigmatic if PTMP1 could be a shear dependent bi-functional cross-linker as postulated previously [9] . Furthermore, other than with integrins [14] , collagen binding is not strictly dependent on the presence of bound metal, with collagen binding being slightly enhanced in the presence of zinc ions in PTMP1 ( Fig. 5e ). It seems feasible that zinc ions have a non-specific stimulating effect on electrostatic interactions between PTMP1 and collagen. Similar effects were observed for another collagen-binding VWA domain protein, Matrilin 3, with collagen-binding properties being also enhanced but not strictly dependent on zinc ions [13] . In the natural context, binding of metal ions to PTMP1 could additionally target other components of the byssus. Since for both observed metal ion binding sites (A1 MIDAS motif and the linker region) three or four complex positions are free or occupied by water molecules, respectively, it is likely that in the native byssus, these positions are occupied by other proteins, for example, the histidine-rich terminal domains of the PreCols, which were also postulated to bind Zn 2+ (ref. 3 ), enabling additional interactions between collagen fibrils and the matrix. In addition, such interactions could be supported by the proline-rich 48-residue N-terminal expansion of PTMP1, which could not be resolved in the crystal structure. Since we could not observe any metal binding to the MIDAS motif of the PTMP1 A2 domain, although it exhibits all prerequisites for efficient coordination, this motif might only be able to coordinate metal ions in the presence of natural coordination partners. It certainly will be a matter for future experiments to reveal the role of metal binding to both MIDAS motifs of PTMP1, and if PTMP1, as postulated earlier, could thereby interconnect byssal collagen molecules or other proteins of the proximal byssus section. It could be shown previously that PTMP1 is a glycoprotein (~11–15 sugar equivalents present) [11] . Each of the two domains comprises one Asn-Xaa-Ser/Thr sequon, a prerequisite for N-linked glycosylation. The respective sequons are located in loops (α1–β2 and α1*–β1*) at the molecule’s surface, suggesting that the glycans observed in the native protein are located at these sites. Alternatively, glycosylation could be linked to the only Thr residue in the flexible N-terminal expansion (T42), as predicted by the NetOGlyc server [34] . There are examples, where glycosylation affects ligand binding of proteins [35] , [36] , [37] . In case of PTMP1 binding to mammalian type-I collagen, it seems not to be affected by glycans, since collagen I binding of recombinantly produced PTMP1 ( K D =0.16 μM) is comparable with that of the native protein ( K D =0.25 μM [11] ). Nevertheless, it is possible that binding of PTMP1 to PreCols in the byssal threads is influenced by glycosylation, since PreCols differ from mammalian collagens concerning amino-acid sequence and structure details. Binding of PTMP1 shows a severe impact on fibril assembly in vitro . Notably, effects of collagen binding/VWA domain containing proteins on collagen assembly were also shown for Matrilin 3 (ref. 38) [38] , albeit the observed effects were not as tremendous as shown for PTMP1, suggesting that collagen binding of proteins with tandem-arranged VWA domains could generally provide a so far undetected control mechanism for collagen/matrix assemblies. In the byssus, PTMP1 is predominantly present in the proximal thread section [11] , with its natural targets being most likely PreCol-P or PreCol-NG rather than PreCol-D. While PreCol-fibrils are more ordered, densely packed and straightly aligned in the distal section [39] , they appear to be more loosely packed and curled in the proximal section [8] , reminiscent to the morphologies of heterologous collagen fibrils assembled in the presence of PTMP1 in vitro . Therefore, PTMP1 might also be involved in controlling collagen assembly and arrangement in the proximal section of a byssus thread. To assign a definite functional role of PTMP1 or a clear contribution of this protein to structure/morphology and mechanical properties of the natural byssus thread is certainly beyond the scope of the current study, although the observed influences of PTMP1 on assembly of heterologous collagens provide a basis for a functional model. The combination of a high structural stability and rigidity of the PTMP1 molecule mediated by its inter-domain linker, its affinity for collagens, and its abundance in the proximal thread section certainly is indicative of a structural and mechanical contribution of PTMP1 to the byssus thread. Furthermore, the impact of matrix proteins like PTMP1 on collagen fibril formation and assembly is obvious when fibres are artificially drawn from purified PreCol proteins [40] , [41] , since these fibres were different from the natural byssal threads with respect to size and mechanical characteristics [10] . Concerning the establishment of collagenous materials with new properties, the in vitro function of PTMP1 might inspire material scientists to adjust morphologies and also mechanical features of reconstituted collagen fibres to be used in different applications, for example, in the generation of gradient materials inspired by the mussel byssus [38] . The possibility to recombinantly produce PTMP1 and other byssal proteins [39] opens the gate for a variety of novel bio-inspired materials based on collagen/matrix assemblies, for example, in tissue engineering [42] . Cloning and expression PTMP1 was cloned and recombinantly produced as described elsewhere (M.H.S., T.S., C.S. and M.G., manuscript in preparation)using the forward primer 5′-GATCTCGGATCCATGGGACATCATGGGGTAATGCC-3′ and the reverse primer 5′-GACTTCGCGGCCGCTTATCCAATGGCTCCTGATCCTTTC-3′. In addition, deletion constructs of PTMP1 were created: ΔNΔC (amino acids 47–442, forward primer: 5′-TAATAGGATCCGAGGAATGCGATGTCCAAGCTG-3′; reverse primer: 5′-TAATTGCGGCCGCTTATGGTTTACAACTCATGCAGGCTA)-3′, A1 (amino acids 47–243; forward primer: 5′-TAATAGGATCCGAGGAATGCGATGTCCAAGCTG-3′; reverse primer: 5′-TGATTGCGGCCGCTTACACTTCACATGCTAGATCGATTACC)-3′, A2 (amino acids 247–439; forward primer: 5′-TGTATGGATCCGACTGTGCCGGACATGCTGATATAGC-3′; reverse primer: 5′-TGATTGCGGCCGCTTAACTCATGCAGGCTAGTTTTACAACATCC-3′). In contrast to the wild-type protein, deletion variants were produced in a 1.5 l Minifors (Infors) bioreactor (fed-batch culture in full medium: 1.62% (w/v) tryptone/peptone from casein, 2.48% (w/v) yeast extract, 15.8 mM potassium dihydrogen phosphate, 40.7 mM ammonium sulphate, 0.75 mM calcium chloride, 4.38 mM magnesium sulphate, supplemented with 35 μg ml −1 kanamycin; base control: 2.5 M sodium hydroxide, acid control: 2.5 M phosphoric acid, foam control: 5% (v/v) Breox FMT 30 antifoam (Cognis), feeding solution: 86% (v/v) glycerol). Cultures were grown at 37 °C to an OD 600 of 40, and gene expression was induced by addition of 0.1 mM IPTG (Roth) at 30 °C. Three hours after induction, cells were harvested by centrifugation. Protein purification After production, PTMP1 and its variants were purified from bacterial inclusion bodies, as described elsewhere (M.H.S., T.S., C.S. and M.G., manuscript in preparation). For experiments, lyophilized proteins were resolubilized in buffer or water, and any insoluble protein was removed by ultracentrifugation (30 min, 186,000 g ). Protein concentrations were determined by ultraviolet spectroscopy using the calculated extinction coefficients (ProtParam, http://www.expasy.org ), which were validated by gravimetric analysis: PTMP1 (15,275 M −1 cm −1 ), ΔNΔC, (9,315 M −1 cm −1 ), A1 (4,595 M −1 cm −1 ), A2 (4,595 M −1 cm −1 ). Protein crystallization and structure solution PTMP1 was crystallized as described elsewhere (M.H.S., T.S., C.S. and M.G., manuscript in preparation), resulting in two crystal forms from initial screening and optimization procedures, respectively, which differed in shape and growth rates. Optionally, improved crystals (M.H.S., T.S., C.S. and M.G., manuscript in preparation) were soaked in cryosolution containing 10 mM magnesium chloride or 50 μM zinc chloride, respectively, for 1 h before freezing. Diffraction data sets were collected at the MX beamline BL14.1 at the BESSY II electron storage ring (Berlin-Adlershof, Germany) operated by the Helmholtz-Zentrum Berlin [43] , with a MX-225 CCD detector (Rayonix, Evanston, USA). Data sets were collected at 100 K and a wavelength of 0.918 Å (crystal form 1 and 2) or 1.283 Å (Zn-soak) over 200° (crystal form 1, Zn-soak) or 130° (crystal form 2) with 1° (crystal form 1 and 2) or 0.5° (Zn-soak) rotation per frame. Indexing, scaling and merging of diffraction data were done with XDS [44] . The initial structure of PTMP1 from a crystal (form 1, box shaped), grown after ~14 days in a JCSG Core Suite I crystallization screen (Qiagen) (M.H.S., T.S., C.S. and M.G., manuscript in preparation), was solved using Patterson searches with Mr Bump [45] . Due to the low-sequence identities (~25%) to VWA proteins with known structures initial phasing attempts by automated molecular replacement failed, but extensive manual searches with various search models, chosen through BLAST searches against the Protein Data Bank employing the ExPASy server ( http://www.expasy.org ), finally yielded individual solutions for the PTMP1 domains A1 (search model PDB-ID 1AOX) and A2 (search model PDB-ID 1QC5). The structure of PTMP1 from improved crystals (form 2, plate shaped, M.H.S., T.S., C.S. and M.G., manuscript in preparation), grown after ~8 days, was solved with molecular replacement using MolRep [46] and the initial PTMP1 structure as a search model. Models were refined using PHENIX [47] , and rebuilding was performed in Coot [48] . For validation of the structures Coot and PROCHECK [49] were used. Structural figures were generated with PyMOL ( http://www.pymol.org ). Surface potential calculations were carried out using APBS [21] . Secondary structure assignment was done with DSSP [50] . CD spectroscopy CD spectra in the far ultraviolet region (190–250 nm) were recorded in a 1-mm cuvette using a Jasco J-815 spectropolarimeter (Jasco) at a scanning speed of 50 nm min −1 , a response time of 2 s and an accumulation of 3–5 single spectra. All spectra were buffer corrected. Thermal stability of the proteins was evaluated by recording the CD signal of 0.2 mg ml −1 protein solutions in 10 mM sodium phosphate, pH 8, at 222 nm with a heating and cooling rate of 60 K h −1 . For analysis of the collagen triple-helical stability, collagen stock solutions of 1 mg ml −1 in 1% acetic acid were diluted fivefold in 50 mM sodium phosphate, and the pH was adjusted to 7.5 with sodium hydroxide. Stability against denaturation with increasing amounts of guanidine hydrochloride was evaluated with 0.2 mg ml −1 protein solutions in 10 mM sodium phosphate, pH 8, by extracting the CD at 222 nm from accumulated spectra of samples incubated overnight. Surface plasmon resonance spectroscopy Collagen type I (Sigma C1809, 0.1 mg ml −1 in 20 mM sodium acetate pH 5) was immobilized on a CM5 sensor chip in a BiacoreX system (GE Healthcare) via amine coupling chemistry according to the manufacturer’s manual (Biacore Surface Sensors Handbook, GE Healthcare). One of the two flow cells (Fc1) was treated with collagen, the other (Fc2) with buffer as a reference. Immobilization resulted in a differential response increase of 8,200 RU, corresponding to 8.2 ng mm −2 immobilized collagen in Fc1. Sensorgrams were recorded at flow rates of 5–20 μl min −1 (typically 10 μl min −1 ). For each experiment, 70 μl of a 10 μM solution of the respective protein dissolved in running buffer (10 mM sodium phosphate, 50 mM sodium chloride, pH 7) were injected, followed by an at least 10-min release phase. After each injection, the chip surface was regenerated using a 70 μl injection of 2 M sodium chloride in running buffer. Sensorgram data (Fc1-Fc2) were analysed using the BIAevaluation 4.1.1 software. Static collagen-binding assay ELISA-like collagen-binding assays were performed as described earlier [11] with several adaptations. Collagens type I–V (Sigma-Aldrich C1809, C3511, C1188, C4407, C5533, C3657) were dissolved in 2% acetic acid by shaking at room temperature overnight. Insoluble contents were removed by centrifugation, and the concentration was adjusted to 1 mg ml −1 in 1% acetic acid. The collagen-resembling triple-helical peptide (PPG) 10 (PeptaNova) was diluted in 10 mM HCl (30 mg ml −1 ). A polyclonal antiserum against full-length PTMP1 was created in a rabbit (Pineda antibody service, Berlin) according to the manufacturer’s standard immunization protocol and tested for specific detection of PTMP1 and its variants in immunoblots. In this study, antiserum of the 150th immunization day was used. Collagen solutions were diluted with 50 mM sodium acetate, pH 5, to a final concentration of 20 μg ml −1 , and 96-well plates were coated with 100 μl of these solutions per well overnight at 4 °C. We used PolySorp plates (Nunc) for our experiments, since they showed negligible background binding, compared with several other assay plates tested. After three washing steps with Tris-buffered saline (TBS), plates were blocked by addition of 300 μl 5% (w/v) BSA for 4 h at room temperature. Subsequently, plates were washed three times with TBS, and solutions of the respective analytes (0–10 μM in TBS, 50 μl per well) were added. After incubation for 2 h, plates were again washed three times with TBS. Then, 50 μl of anti-PTMP1 serum (1:10,000 dilution in TBS) was added and incubated for 45 min. Unbound antibodies were removed by three washing steps with TBS-T (TBS containing 0.05% (v/v) Tween 20). Subsequently, 50 μl of a horseradish peroxidase-conjugated anti-rabbit antibody (Sigma-Aldrich) was added (1:20,000 dilution in TBS) and incubated for 45 min. After three washes with TBS-T and an additional washing step with TBS, complexes were detected using 50 μl 3,3′,5,5′-tetramethylbenzidin as a substrate (0.1 mg ml −1 3,3′,5,5′-tetramethylbenzidin in 100 mM sodium acetate, 4 mM citric acid, 4.7 mM hydrogen peroxide). The reaction was stopped after 5 min with 50 μl of 0.5 M sulphuric acid, and colour development was measured at 450 nm in an automated plate reader by accumulating five single reads. As a control, binding of primary and secondary antibodies to the collagens was tested, as well as the binding (without collagens) of the respective antibodies and analytes to blocked and unblocked plates. Different blocking reagents, up to 1% BSA in the analyte solutions and Tween 20 concentrations up to 1% (v/v) in the washing buffers, were tested. For data analysis, the absorption was plotted against the analyte concentration. Apparent dissociation constants were obtained from nonlinear regression of the data (Origin 8.1, OriginLab) according to a one-site binding model employing the Michaelis–Menten equation [51] . The influence of divalent metal ions on collagen binding of PTMP1 and its variants was tested by addition of 0.1–10 mM MgCl 2 , CaCl 2 , MnCl 2 and ZnCl 2 , respectively, to the analyte solutions. Microscopic analysis of collagen fibrils Collagen fibrils were assembled from collagen type I (Sigma C1809, C3511) according to Williams et al. [29] by 10-fold dilution of the 1 mg ml −1 collagen stock solution (1% acetic acid) into 10 mM sodium phosphate pH 8, 150 mM sodium chloride, adjusting the pH with sodium hydroxide. 0.1 mg ml −1 PTMP1 were added from a highly concentrated buffered stock solution, and samples were incubated at room temperature overnight. For TEM, samples were diluted 10-fold into a MilliQ-filtered water droplet, and a Formvar-coated copper TEM grid was immediately placed on top. After incubation for 1 min, the grid was washed twice with MilliQ-filtered water and stained for 30 s with a saturated solution of uranyl acetate. After an additional washing step with water, the grids were dried, and TEM images were recorded on a JEM-2100 transmission electron microscope (JEOL), operated at 80 kV and equipped with an ES500W Erlangshen camera (Gatan). For AFM, samples were diluted 2–10-fold with MilliQ-filtered water and incubated for 3 min on a freshly cleaved muscovite (mica) surface. After three washing steps with MilliQ-filtered water, samples were air dried. Tapping mode AFM images were recorded using OMCL-AC160TS-W2 cantilevers (Olympus) using a dimension 3,100 scanning force microscope, equipped with a nanoscope IV controller and a closed-loop XY tip scanner (Veeco). Accession codes : Coordinates and diffraction data have been deposited with the Protein Data Bank ( http://www.pdb.org ): crystal form I (entry ID 4CN8 ), crystal form II ( 4CNB ), Zn 2+ complex ( 4CN9 ). How to cite this article : Suhre, M. H. et al. Structural and functional features of a collagen-binding matrix protein from the mussel byssus. Nat. Commun. 5:3392 doi: 10.1038/ncomms4392 (2014).